Dark acoustic metamaterials as super absorbers for low-frequency sound The attenuation of low-frequency sound has been a challenging task because the intrinsic dissipation of materials is inherently weak in this regime. Here we present a thin-film acoustic metamaterial, comprising an elastic membrane decorated with asymmetric rigid platelets that aims to totally absorb low-frequency airborne sound at selective resonance frequencies ranging from 100–1,000 Hz. Our samples can reach almost unity absorption at frequencies where the relevant sound wavelength in air is three orders of magnitude larger than the membrane thickness. At resonances, the flapping motion of the rigid platelets leads naturally to large elastic curvature energy density at their perimeter regions. As the flapping motions couple only minimally to the radiation modes, the overall energy density in the membrane can be two-to-three orders of magnitude larger than the incident wave energy density at low frequencies, forming in essence an open cavity. The attenuation of low-frequency sound has been a challenging task because the dynamics of dissipative systems are generally governed by the rules of linear response, which dictate the frictional forces and fluxes to be both linearly proportional to the rates. It follows that the dissipative power is quadratic in rates, thereby accounting for the inherently weak absorption of low-frequency sound waves by homogeneous materials. To enhance the dissipation at low frequencies, it is usually necessary to increase the energy density inside the relevant material, for example, through resonances. However, in an open system radiation coupling to resonances is an alternative that can be effective in reducing dissipation. Although the advent of acoustic metamaterials has broadened the realm of possible material characteristics [1] , [2] , [3] , [4] , [5] , [6] , [7] , [8] , [9] , [10] , [11] , [12] , [13] , [14] , [15] , [16] , [17] , [18] , [19] , [20] , [21] , [22] , [23] , [24] , as yet, there are no specific resonant structures targeting the efficient and subwavelength absorption of low-frequency sound. In contrast, various electromagnetic metamaterials designed for absorption have been proposed [25] , [26] , [27] , [28] , [29] , [30] , [31] , [32] , [33] , [34] , and an 'optical black hole' has been realized by using metamaterials to guide the incident wave into a lossy core [35] , [36] . In this work, we show that by using thin elastic membranes decorated with designed patterns of rigid platelets, the resulting acoustic metamaterials can absorb 86% of the acoustic waves at ∼ 170 Hz, with two layers absorbing 99% at the lowest frequency resonant mode as well as at higher frequency modes. The sample is thus acoustically 'dark', at those frequencies. Finite element simulations of the resonant mode patterns and frequencies are in excellent agreement with the experiments. In particular, the measured displacement profiles of the resonant modes show discontinuities in the slope around the platelet perimeters, implying significantly enhanced curvature energy is concentrated in these small volumes, which are minimally coupled to the radiation modes. This thereby gives rise to strong absorption similar to a cavity system, even though the system is geometrically open. This is characterized by the fact that at resonances, the overall energy density in the system can be two-to-three orders of magnitude larger than the incident wave's energy density. Sample constructs and absorption coefficient measurements We first focus on a relatively simple, proof-of-principle structure, denoted Sample A. In Fig. 1a , we show a photo of the unit cell used in the experiment, comprising a rectangular elastic membrane that is 31 mm by 15 mm and 0.2 mm thick. The elastic membrane was fixed by a relatively rigid grid, decorated with two semi-circular iron platelets with a radius of 6 mm and thickness of 1 mm. The iron platelets are purposely made to be asymmetrical so as to induce flapping motion, as seen below. Here the sample lies in the x – y plane, with the two platelets separated along the x axis. Acoustic waves are incident along the z direction. This simple cell is used to understand the relevant mechanism and to compare with theoretical predictions. 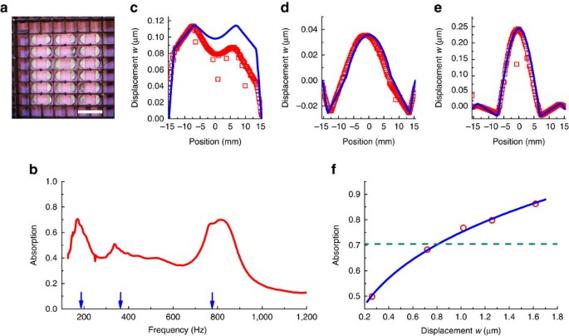Figure 1: Absorption coefficient and displacement profiles of sample A. (a) Photo of Sample A. The scale bar is 30 mm. (b) The measured absorption coefficient (red curve) and the positions of the absorption peak frequencies predicted by finite-element simulations (blue arrows). There are three absorption peaks located at 172, 340 and 813 Hz. (c), (d), (e) The cross-sectional profiles ofz-displacement,w, along thexaxis of the unit cell for each of the three resonances. The measuredz-displacement profiles by laser vibrometer (red squares) and the finite-element simulation results (blue curves) around 172, 340 and 813 Hz are shown in (c), (d) and (e), respectively. The straight sections (7.5 mm≤|x|≤13.5 mm) of the profile indicate the positions of the platelets, which may be regarded as rigid. (f) Red circles denote the experimentally measured absorption coefficient and the magnitude of the membrane displacementwat 172 Hz when the distance between the membrane and the aluminum reflector was varied from 7 to 42 mm with 7 mm steps. The blue solid curve is a guide to the eye. The dashed line denotes the absorption level when the aluminum reflector is removed, that is, when the distance between the membrane and the aluminum reflector tends to infinity. Figure 1: Absorption coefficient and displacement profiles of sample A. ( a ) Photo of Sample A. The scale bar is 30 mm. ( b ) The measured absorption coefficient (red curve) and the positions of the absorption peak frequencies predicted by finite-element simulations (blue arrows). There are three absorption peaks located at 172, 340 and 813 Hz. ( c ), ( d ), ( e ) The cross-sectional profiles of z -displacement, w , along the x axis of the unit cell for each of the three resonances. The measured z -displacement profiles by laser vibrometer (red squares) and the finite-element simulation results (blue curves) around 172, 340 and 813 Hz are shown in ( c ), ( d ) and ( e ), respectively. The straight sections (7.5 mm≤| x |≤13.5 mm) of the profile indicate the positions of the platelets, which may be regarded as rigid. ( f ) Red circles denote the experimentally measured absorption coefficient and the magnitude of the membrane displacement w at 172 Hz when the distance between the membrane and the aluminum reflector was varied from 7 to 42 mm with 7 mm steps. The blue solid curve is a guide to the eye. The dashed line denotes the absorption level when the aluminum reflector is removed, that is, when the distance between the membrane and the aluminum reflector tends to infinity. Full size image Another type of unit cell, denoted Sample B, is 159 mm by 15 mm and comprises 8 identical platelets decorated symmetrically as two 4-platelet arrays (with 15 mm separation between the neighbouring platelets) facing each other with a central gap of 32 mm. Sample B is used to attain near-unity absorption of the low-frequency sound at multiple frequencies. The measured absorption as a function of frequency for Sample A is shown in Fig. 1b , where it can be seen that there are 3 absorption peaks around 172, 340, and 813 Hz. But perhaps the most surprising is the absorption peak at 172 Hz, at which more than 70% of the incident acoustic wave energy has been dissipated. This is a very high value by such a 200-μm membrane, given that the wavelength in air at such a low frequency is about 2 m. Below we show this phenomenon to arise directly from the profiles of the membrane resonances. In Fig. 1b we also indicate the calculated absorption peak frequencies by blue arrows. The Young's modulus and Poisson's ratio for the rubber membrane are 1.9×10 6 Pa and 0.48, respectively, which had been measured experimentally by Damping Technologies (Methods). The imaginary part of the Young's modulus is taken to be in the form Im( E )≡ ωχ 0 , where ω is the angular frequency and χ 0 =7.96×10 2 Pa s is obtained by fitting to the absorption (Methods). Many eigenmodes are found in the simulations. Out of these, we select the ones that are left–right symmetric, because the anti-symmetric ones would not couple to the normally incident plane wave. The resulting absorption peak frequencies are located at 190, 346 and 712 Hz, respectively (indicated by the blue arrows in Fig. 1b ). They are seen to agree very well with the observed peak frequencies. Out-of-plane displacement profiles measurement In Fig. 1c–e , we show the cross-sectional profile of the z -displacement w along the x axis, within the unit cell for the three absorption peak frequencies. Red squares denote the experimental measured data by laser vibrometer, whereas the blue curves are the finite-element simulation results. Excellent agreement is seen. But the most prominent feature of the profiles is that although the z -displacement w is continuous at the perimeters of the platelets (whose positions are indicated by the straight sections of the curves where the curvature is zero), there exists a sharp discontinuity in the first-order spatial derivative of w normal to the perimeter. For the low-frequency resonance, this discontinuity is caused by the flapping motion of the two semicircular platelets that is symmetric with respect to the x axis, whereas, for the 712 Hz resonance, it is caused by the large vibration of the central membrane region, with the two platelets acting as anchors. The intermediate frequency mode is also a flapping mode, but with the two ends of each wing in opposite phase. Tuning the sample impedance In Fig. 1f , we show the results of further tuning the impedance of the membrane by placing an aluminum reflector at various near-field distances behind the membrane. Here the absorption at 172 Hz is plotted as a function of the measured maximum normal displacement of the membrane, for an incident wave with pressure modulation amplitude of 0.3 Pa. Each symbol (open circle) indicates a distance of separation between the membrane and the reflector, varying from 7 to 42 mm in steps of 7 mm each. It is seen that adding an air cushion can enhance the absorption, up to 86% at a separation of 42 mm. That is roughly 2% of the wavelength. However, moving the reflector further will eventually reduce the absorption to the value without the reflector, as indicated by the dashed line. Absorption frequency tunability The characters of the membrane eigenmodes dictate the manner under which their resonance frequencies are tunable: while for the flapping mode the frequency is shown to decrease when the platelet mass is increased, the membrane vibration mode frequency can be increased or decreased by varying the distance of separation between the two semicircular platelets. More specifically, in Fig. 2a,b , we show the tunability of the absorption peaks at 172 Hz and 813 Hz, respectively. The message is essentially that the low-frequency peak varies as where M denotes the mass of a single platelet (whereas the high-frequency peak is only minimally affected by varying M ), and the high-frequency peak varies as 1/ L , with L being the separation between the two platelets (whereas the low-frequency peak is only minimally affected by varying L ). It is seen that the measured data (red circles) agree very well with the simulation results (blue triangles). 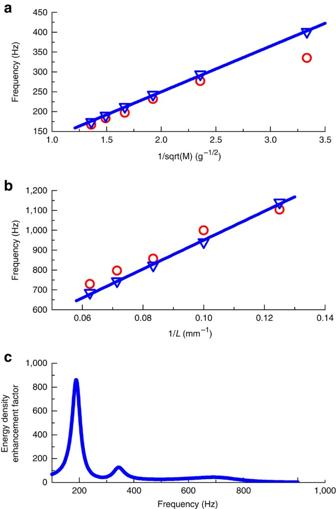Figure 2: Absorption frequency tunability and the EDEF. (a) The flapping mode frequency plotted as a function of each platelet's massM. The red circles denote the experimental data and blue triangles the simulation results. It can be seen that the low-frequency absorption peak (172 Hz) in Fig. 1b varies as the inverse of the square root ofM. The blue solid line is to guide the eye. (b) The membrane vibration mode frequency (813 Hz in Fig. 1b) as a function of the separationLbetween the two platelets. The red circles denote the experimental data and blue triangles the simulation results. It can be seen that the high-frequency absorption peak (813 Hz) in Fig. 1b varies as the inverse of the separationL. The blue solid line is to guide the eye. (c) The EDEF for Sample A, plotted as a function of frequency. The maximum values of EDEF occur at the same frequencies as the absorption peaks. The relatively smaller values of EDEF at higher frequencies are noted to be compensated by theω2dependence of the absorption coefficient (see equation (2)). Figure 2: Absorption frequency tunability and the EDEF. ( a ) The flapping mode frequency plotted as a function of each platelet's mass M . The red circles denote the experimental data and blue triangles the simulation results. It can be seen that the low-frequency absorption peak (172 Hz) in Fig. 1b varies as the inverse of the square root of M . The blue solid line is to guide the eye. ( b ) The membrane vibration mode frequency (813 Hz in Fig. 1b) as a function of the separation L between the two platelets. The red circles denote the experimental data and blue triangles the simulation results. It can be seen that the high-frequency absorption peak (813 Hz) in Fig. 1b varies as the inverse of the separation L . The blue solid line is to guide the eye. ( c ) The EDEF for Sample A, plotted as a function of frequency. The maximum values of EDEF occur at the same frequencies as the absorption peaks. The relatively smaller values of EDEF at higher frequencies are noted to be compensated by the ω 2 dependence of the absorption coefficient (see equation (2)). Full size image Elastic energy density via finite-element simulations To understand the strong absorption, it is useful to consider the bending wave (or flexural wave) of a thin solid elastic membrane satisfying the biharmonic equation [37] : where is the flexural rigidity and h is the thickness of the membrane, with ρ , E , and v being the mass density, Young's modulus, and Poisson's ratio, respectively. The corresponding elastic curvature energy per unit area is given by [37] , [38] As Ω is a function of the second-order spatial derivatives of w , when the first-order derivative of w is discontinuous across the edge boundary, it is easy to infer that the areal energy density Ω should have a very large value within the perimeter region (divergent in the limit of a thin shell). Moreover, as the second derivative is quadratic, the integrated value of the total potential energy must also be very large. In the limit of small h , the vibrational modes of our system may be regarded as a weak-form solution of the shell model, in the sense that, although the biharmonic equation is not satisfied at the perimeter of the platelets (because the higher order derivatives do not exist), besides this set of points with measure zero, the solution is still a minimizer of the relevant Lagrangian. The predicted large value of Ω within the perimeter region is easily verified as shown in Fig. 3 , where we plot the elastic potential energy density U obtained from the COMSOL simulations ( Fig. 3a , where the colour is assigned according to a logarithmic scale, base 10) and displacement w ( Fig. 3b ) distribution within the x-y plane (that is, the mid-plane of the membrane) around three absorption peak frequencies: 190, 346, and 712 Hz (from top to bottom). The energy density in the perimeter region is seen to be larger than that in other regions by 3–4 orders of magnitude. There are also high-energy density regions at the upper and lower edges of the unit cell, where the membrane is clamped. In our simulations, the integrated energy density U within the perimeter region accounts for 98% (190 Hz), 87% (346 Hz), and 82% (712 Hz) of the total elastic energy in the whole system. As the local dissipation is proportional to the product of energy density with dissipation coefficient, the large multiplying effect implied by the huge energy density can mean very substantial absorption for the system as a whole. This fact is also reflected in the strain distribution around the three absorption peak frequencies, as shown in Fig. 3c . It is found that the strain in the perimeter region, on the order of 10 −3 –10 −4 , is much larger than that in the other parts of the membrane by at least 1–2 orders of magnitude. 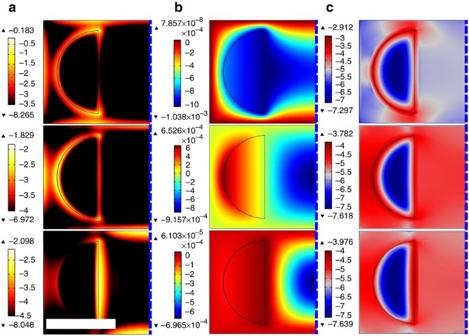Figure 3: Elastic energy density distribution within Sample A. (a) The calculated distributions of the elastic potential energy density within thex–yplane. (b) The calculated normal displacementwwithin thex–yplane. (c) The calculated distribution of the trace of the strain tensorɛ=ɛxx+ɛyy+ɛzzwithin thex–yplane. In (a), (b), and (c), the three rows, from top to bottom, are for the three absorption peak frequencies of 190 Hz, 346 Hz, and 712 Hz, respectively. In (a) and (c), the colour bars indicate the relative magnitudes of the quantities in question, with the numbers shown to be the logarithms of the magnitudes, base 10. In (b), the colour bar scale is linear. As these modes are symmetric with respect to thexcoordinate, we plot only the left half for better resolution. The straight dashed blue lines indicate the mirroring planes. The scale bar is 10 mm. Figure 3: Elastic energy density distribution within Sample A. ( a ) The calculated distributions of the elastic potential energy density within the x – y plane. ( b ) The calculated normal displacement w within the x – y plane. ( c ) The calculated distribution of the trace of the strain tensor ɛ = ɛ xx + ɛ yy + ɛ zz within the x – y plane. In ( a ), ( b ), and ( c ), the three rows, from top to bottom, are for the three absorption peak frequencies of 190 Hz, 346 Hz, and 712 Hz, respectively. In ( a ) and ( c ), the colour bars indicate the relative magnitudes of the quantities in question, with the numbers shown to be the logarithms of the magnitudes, base 10. In ( b ), the colour bar scale is linear. As these modes are symmetric with respect to the x coordinate, we plot only the left half for better resolution. The straight dashed blue lines indicate the mirroring planes. The scale bar is 10 mm. Full size image Energy density enhancement factor In accordance with our metamaterial being highly absorptive, our sample may be characterized by an effective parameter—the energy density enhancement factor (EDEF)—defined to be the ratio of the average energy inside the sample to the energy density of the incident wave. As discussed previously, the physical mechanism of such a high absorption is the flapping motion of the metallic platelets, attendant with a very high elastic curvature energy density within the perimeter region of the platelets. A plot of the calculated EDEF for Sample A as a function of frequency, ranging from 100–1,000 at resonances, is shown in Fig. 2c . It is seen that the value of EDEF ranges from 100–1,000 at resonances. For absorption, the relatively smaller values of EDEF at higher frequencies are compensated by the ω 2 dependence of the absorption coefficient (see equation (2) below). Thus, our samples may be regarded as an open cavity, a concept that is further elaborated in the Discussion. Achieving near-unity absorption As the high curvature energy density is mostly confined in the perimeter regions of the platelets and the edges of the unit cell, we may attain better absorption by further tweaking the unit cell structure. Compared with Sample A, the unit cell of Sample B has more platelets and longer edges ( Fig. 4a ), while its eigenmodes mostly remain unchanged in character due to the similar layout (see Supplementary Fig. S1 for experimental data in favour of this conclusion). Therefore, Sample B should be similar to Sample A but should display better absorption performance. 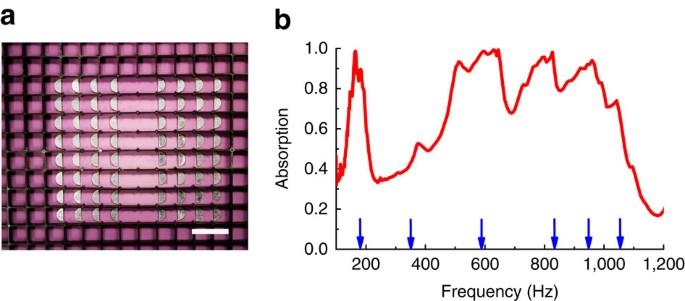Figure 4: Absorption coefficient of sample B. (a) Photo of Sample B. The scale bar is 30 mm. (b) The red curve indicates the experimentally measured absorption coefficient for two layers of Sample B with an aluminum reflector placed 28 mm behind the second layer. The distance between the first and second layers is also 28 mm. The absorption peaks are located at 164, 376, 511, 645, 827 and 960 Hz. Blue arrows indicate the positions of the absorption peak frequencies predicted by finite-element simulations. Good agreement is seen. Figure 4: Absorption coefficient of sample B. ( a ) Photo of Sample B. The scale bar is 30 mm. ( b ) The red curve indicates the experimentally measured absorption coefficient for two layers of Sample B with an aluminum reflector placed 28 mm behind the second layer. The distance between the first and second layers is also 28 mm. The absorption peaks are located at 164, 376, 511, 645, 827 and 960 Hz. Blue arrows indicate the positions of the absorption peak frequencies predicted by finite-element simulations. Good agreement is seen. Full size image As shown in Fig. 4b , that is indeed the case. In our measurements, we have two layers of Sample B, and tune the impedance of the system by placing an aluminum reflector 28 mm behind the second layer. The distance between the first and second layers was also 28 mm. It can be seen that there are many absorption peaks around 164, 376, 511, 645, 827, and 960 Hz. The absorption peaks at 164 Hz and 645 Hz are seen to be ∼ 99%. By using COMSOL, we have also calculated the absorption peak frequencies for a single layer of Sample B. They are located around 170, 321, 546, 771, 872 and 969 Hz, respectively. These are indicated by blue arrows in Fig. 4b . Reasonably good agreement with the experimental values is seen, with no adjustable parameters. Absorption calculation In accordance with the Poynting's theorem for elastic waves [39] , the dissipated power within the membrane can be calculated as where U is the elastic energy density in the sample. Absorption is defined as Q /( PS ), where P = p 2 /( ρc ) denotes the Poynting's vector for the incident acoustic wave and S is membrane's area, with p , ρ and c being the pressure amplitude, mass density and sound velocity of air, respectively. With the previously given parameter values, the absorption at the three resonant frequencies of Sample A (in order of increasing frequency) is calculated to be 60, 29 and 43%, respectively. It is noted that the calculated values reproduce the relative pattern of the three absorption peaks, although they are smaller than the experimental values by ∼ 10–20%. This discrepancy is attributed to the imperfection in the symmetry of the sample, whereby a multitude of asymmetric vibrational eigenfunctions can be excited by the normally incident plane wave. Together with the width of these modes, they can effectively contribute to a level of background absorption not accounted for in the simulations. In fact, the excitation of asymmetric vibrational mode was experimentally observed, shown in Supplementary Fig. S1 . Difference with the reflective metamaterial To contrast with our previous membrane-type metamaterials that exhibit near-total reflection at an anti-resonance frequency [2] , [3] , here we describe briefly the mechanism of such reflective metamaterials as well as present their measured absorption performance. Strong reflection of sound can occur at a frequency in-between two neighbouring resonant (eigenmode) frequencies. That is, while at the resonant eigenmode frequency the excitation of the eigenmodes can lead to transmission peaks, at the anti-resonance frequency the out-of-phase hybridization of two nearby eigenmodes leads to a near-total decoupling of the membrane structure from the radiation modes. This turns out to also coincide with a divergent resonance-like behaviour of the dynamic mass density [2] . Near-total reflection of the acoustic wave is thereby the consequence at the anti-resonance frequency. Because the structure is completely decoupled from the acoustic wave at the anti-resonance frequency, the absorption is naturally very low as shown in Fig. 5a near 450 Hz (a sharp transmission dip can be seen at this frequency in the logarithmic scale). But, even at the resonant frequencies, we note that the absorption coefficient for this type of metamaterial is still low, barely reaching 45% at the relatively high frequency of 913 Hz, not even close to what we have achieved with the dark acoustic metamaterials. This is attributed to the relatively strong coupling to the radiation modes caused by the piston-like motion of membrane that can lead to high transmission (0.88 at 251 Hz, 0.63 at 913 Hz). 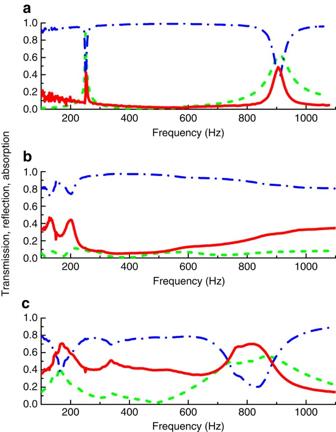Figure 5: Difference between the reflective and absorptive metamaterials. (a) Measured transmissionT(green dashed curve), reflectionR(blue dot-dashed curve) and absorptionA=1−R2−T2(red solid curve) for a one-layer sample of reflective metamaterial (see ref.2for details) comprising a circular elastic membrane fixed by a rigid grid and with one circular disk attached to the centre. It is seen that at the anti-resonance frequency of 450 Hz, where the membrane is nearly totally reflective (a sharp dip in transmission, at that frequency, is visible in the logarithmic scale), the absorption is very low. Even at the resonance frequencies, the two peaks of absorption are just over 40%, much smaller than that of Sample A, shown in (c). (b) The corresponding experimental data for a five-layer sample of reflective metamaterial (see ref.3for details) sandwiched by two soft panels with holes (for the purpose of enhancing the absorption), with each layer comprising a matrix of square elastic membranes fixed by a rigid grid, and decorated with multiple circular disks with different weights (for the purpose of inducing multiple resonances and hence effecting a nearly broad-band reflective functionality between 100 and 1,000 Hz). The overall absorption is seen to be small as compared with that of Sample A, shown in (c). (c) The corresponding experimental data for the one-layer Sample A, without a back reflector. The overall absorption is high (around 40%). In particular, at the resonance frequency of 172 Hz, the peak absorption can reach 70%. Figure 5: Difference between the reflective and absorptive metamaterials. ( a ) Measured transmission T (green dashed curve), reflection R (blue dot-dashed curve) and absorption A =1− R 2 − T 2 (red solid curve) for a one-layer sample of reflective metamaterial (see ref. 2 for details) comprising a circular elastic membrane fixed by a rigid grid and with one circular disk attached to the centre. It is seen that at the anti-resonance frequency of 450 Hz, where the membrane is nearly totally reflective (a sharp dip in transmission, at that frequency, is visible in the logarithmic scale), the absorption is very low. Even at the resonance frequencies, the two peaks of absorption are just over 40%, much smaller than that of Sample A, shown in ( c ). ( b ) The corresponding experimental data for a five-layer sample of reflective metamaterial (see ref. 3 for details) sandwiched by two soft panels with holes (for the purpose of enhancing the absorption), with each layer comprising a matrix of square elastic membranes fixed by a rigid grid, and decorated with multiple circular disks with different weights (for the purpose of inducing multiple resonances and hence effecting a nearly broad-band reflective functionality between 100 and 1,000 Hz). The overall absorption is seen to be small as compared with that of Sample A, shown in ( c ). ( c ) The corresponding experimental data for the one-layer Sample A, without a back reflector. The overall absorption is high (around 40%). In particular, at the resonance frequency of 172 Hz, the peak absorption can reach 70%. Full size image Even for a five-layer sample [3] , the averaged absorption coefficient is a mere 0.22, with maximum value not surpassing 0.45, as shown in Fig. 5b . And, we must emphasize that besides the large number of membrane layers, this sample was also sandwiched by two soft panels with holes, with the purpose of enhancing the absorption. Therefore, even with these efforts, this panel's absorption performance is still way below our dark acoustic metamaterials. To contrast with the reflection panels, in Fig. 5c we show the transmittance and reflectance data (together with the absorption) of our Sample A. It is seen that with this single-layer sample the absorption can already exceed that of the five-layer sample by a significant amount. Such a large difference is due to the fact that the high energy density regions in our super-absorptive acoustic metamaterial couple minimally with the radiation modes, thereby behaving as an open cavity. Absorption under oblique incidence As mentioned earlier, there are many eigenmodes in the system that are decoupled from the normally incident wave owing to its left–right symmetry. To explore the consequence when such symmetry is broken, we have also carried out measurements on Sample B under oblique incidence. The measured data and simulation results, discussed and presented in Supplementary Figs S2–S4 and the Supplementary Discussion , indicate qualitative similarity up to 60°, at which angle the frequency ranges of 650–950 Hz and 1,000–1,200 Hz exhibit a pronounced increase in absorption. Thus, the overall performance of the dark acoustic metamaterials does not deteriorate under a broad range of incident angles but may even improve within certain frequency regimes. In a conventional open system, high energy density is equally likely to be radiated, via transmitted and reflected waves, as to be absorbed. We wish to point out that in the present case, the small volumes in which the elastic energy is concentrated may be regarded as an open cavity in which the lateral confinement in the plane of the membrane is supplemented by the confinement in the normal direction, owing to the fact that the relative motion between the platelets and the membrane contributes only minimally to the average normal displacement of the membrane. Hence, from the dispersion relation for the waves in air, where k || ( k ⊥ ) denotes the component of the wave vector being parallel (perpendicular) to the membrane plane and λ is the wavelength in air, it can be seen that the relative motions between the platelets and the membrane must be on a scale smaller than the sample size d << λ . Therefore, these motions can only couple to the evanescent waves as the relevant Only the average normal displacement of the membrane, corresponding to the piston-like motion, would have k || components that are peaked at zero and hence can radiate. But the high energy density regions (especially those associated with the flapping modes), owing to their small lateral dimensions, contribute minimally to the average component of the normal displacement. We have demonstrated that the effect of very large curvature energy density at the perimeter of the platelets, in conjunction with its confinement effect, can be particularly effective for subwavelength low-frequency acoustic absorption. As the membrane system has also been shown to be effective in totally reflecting low-frequency sound [2] , [3] , together they can constitute a system of low-frequency sound manipulation with broad potential applications. In particular, lowering the cabin noise in airliners and ships, tuning the acoustic quality of music halls, and environmental noise abatement along highways and railways are some promising examples. Young's modulus and Poisson's ratio of the membrane In the experiments, the membrane is made of silicone rubber Silastic 3133. The Young's modulus and the Poisson's ratio of the membrane were measured by Damping Technologies. The measurement was performed in the ASTM E-756 sandwich beam configuration, where the dynamic mechanical properties of the membrane were obtained from the measured difference between the steel base beam (without membrane) properties and the properties of the assembled sandwich beam test article (with the membrane sandwiched in the core of the beam). In the measurement, the shear modulus ( μ ) data of the membrane at several discrete frequencies could be obtained. The Poisson ratio ( ν ) of the membrane was found to be around 0.48. Therefore, according to the relation between different elastic parameters, we obtain the Young's modulus ( E ) at those discrete frequencies, shown as red circles in Fig. 6 . For our material, the measured E varies from 1.2×10 6 Pa to 2.6×10 6 Pa within the relevant frequency range. We have chosen to use a frequency-independent value of the Young's modulus E =1.9×10 6 Pa (shown as the dashed line in Fig. 6 ) so as to simplify the model. 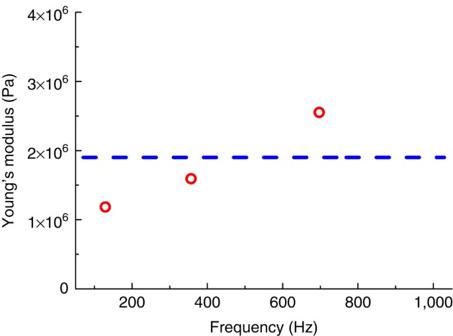Figure 6: Young's modulus of the thin-film membrane. Red circles denote the measured Young's modulusEat several frequencies. Blue dashed curves denote the average value, 1.9×106Pa, within the relevant frequency range. Figure 6: Young's modulus of the thin-film membrane. Red circles denote the measured Young's modulus E at several frequencies. Blue dashed curves denote the average value, 1.9×10 6 Pa, within the relevant frequency range. Full size image Experimental set-up Measurements of the absorption coefficients shown in Figs 1b,f ; 4b and 5 were conducted in modified impedance tube apparatus [40] comprising two Brüel & Kjær Type-4206 impedance tubes with the sample sandwiched in between. The front tube has a loud speaker at one end to generate a plane wave. Two sensors were installed in the front tube to sense the incident and reflected waves, thereby obtaining both the reflection amplitude and phase. The third sensor in the back tube (which is terminated with an anechoic sponge) senses the transmitted wave, to obtain the transmission amplitude and phase. The anechoic sponge has a length of 25 cm, sufficient to ensure complete absorption of the transmitted wave behind the third sensor. The signals from the three sensors are sufficient to resolve the transmitted and reflected wave amplitudes, in conjunction with their phases. The absorption coefficient was evaluated as A =1− R 2 − T 2 , with R and T being the measured reflection and transmission coefficients, respectively. The absorption measurements were calibrated to be accurate by using materials of known dissipation. For the oblique incidence, wedges with designated angles are machined out of aluminum to introduce angles between the axis of the impedance tube and the sample. An aluminum plate is fixed behind the sample to eliminate transmission. Therefore, the sensor on the transmission side is not needed for oblique measurement of absorption. A photo of the set-up is shown in Supplementary Fig. S2 . The cross-sectional profiles of the z -direction displacement shown in Fig. 1c–e were obtained by using the laser vibrometer (Type No. Graphtec AT500-05) to scan the Sample A along the x axis, within the unit cell around the three absorption peak frequencies. Theory and simulations The numerical simulation results shown in Figs 1b–e , 2 , 3 and 4b were prepared using COMSOL MULTIPHYSICS, a finite-element analysis and solver software package. In the simulations, the edges of the rectangular membrane are fixed. An initial stress in the membrane, was used in the calculation as the tunable parameter to fit the data. The mass density, Young's modulus and Poisson's ratio for the rubber membrane are 980 kg m −3 , 1.9×10 6 Pa, and 0.48, respectively. The mass density, Young's modulus and Poisson's ratio for the iron platelets are 7,870 kg m −3 , 2×10 11 Pa, and 0.30, respectively. Standard values for air, that is, ρ =1.29 kg m −3 , ambient pressure of 1 atm, and speed of sound in air of c =340 m s −1 , were used. Radiation boundary conditions were used at the input and output planes of the air domains in the simulations. How to cite this article: Mei, J. et al . Dark acoustic metamaterials as super absorbers for low-frequency sound. Nat. Commun. 3:756 doi: 10.1038/ncomms1758 (2012).